Semi-permeable coatings fabricated from comb-polymers efficiently protect proteinsin vivo In comparison to neutral linear polymers, functional and architecturally complex (that is, non-linear) polymers offer distinct opportunities for enhancing the properties and performance of therapeutic proteins. However, understanding how to harness these parameters is challenging, and studies that capitalize on them in vivo are scarce. Here we present an in vivo demonstration that modification of a protein with a polymer of appropriate architecture can impart low immunogenicity, with a commensurably low loss of therapeutic activity. These combined properties are inaccessible by conventional strategies using linear polymers. For the model protein L -asparaginase, a comb-polymer bio-conjugate significantly outperformed the linear polymer control in terms of lower immune response and more sustained bioactivity. The semi-permeability characteristics of the coatings are consistent with the phase diagram of the polymer, which will facilitate the application of this strategy to other proteins and with other therapeutic models. Many advances in biotechnology can be linked to the development of robust methods for producing well-defined functional polymers. For instance, anionic polymerization has yielded one of the first well-defined linear polymers, α-methoxy-poly(ethylene glycol) (mPEG), variants of which have profoundly marked the pharmaceutical sector as protective coatings for protein drugs [1] , [2] , [3] . Controlled radical polymerization has also permitted the design of numerous macromolecular drugs, polymer–drug and polymer–protein conjugates [4] . The state-of-the-art of tailored polymer synthesis is currently evolving, the controlled polymerization of functional monomers has become commonplace [5] and new tools for preparing polymers with defined sequences and topologies continue to emerge [6] , [7] . In comparison to neutral linear polymers, functional and architecturally complex, that is, nonlinear, polymers offer numerous additional opportunities for enhancing the potential of therapeutic proteins, but have only recently drawn attention in therapeutics. Maynard and co-workers have shown that basic fibroblast growth factor could be stabilized by covalent conjugation with a heparin-mimicking polymer containing styrene sulfonate and oligo(ethylene glycol) monomethyl ether methacrylate (OEGMA) units [8] . The conjugate was stable to a variety of environmentally and therapeutically relevant stressors such as heat, acid, storage and proteases. Keefe and Jiang showed how a poly(zwitterionic) polymer grafted to α-chymotrypsin strongly stabilized the latter, even towards strong denaturants, via non-covalent interactions between the polymer and the protein [9] . Unfortunately, in vivo studies are scarce. Leroux and co-workers recently demonstrated that the functionality of different polymers grafted to proline-specific endopeptidases could be manipulated to stabilize and alter the dwell time of orally administered enzymes at different locations in the gastrointestinal tract [10] . Such studies are crucial because trends and observations made in vitro often do not correlate with in vivo observations [11] . This is in part due to the complex and potentially unpredictable nature of the interactions between the conjugate and components of the body. Our group has recently discovered that comb-shaped poly-OEGMA (pOEGMA) chains with well-defined aspect ratios could generate a molecular sieving effect in vitro when grafted to the surface of a protein [12] . Within a certain regime of polymer characteristics, small molecules could easily diffuse through the coating towards the catalytic site of an enzyme (that is, maintaining high activity), whereas macromolecules were simultaneously blocked. This selective permeability phenomenon, which cannot be emulated with linear mPEG, could be of exceptional value for reducing the immunogenicity of recombinant, non-human-derived therapeutic enzymes without hindering catalytic processing of small molecules. One protein that falls into this category is L -asparaginase (ASNase), an enzyme that is used for treating acute lymphoblastic leukaemia. This protein was one of the first to be modified with mPEG because of its propensity to cause severe hypersensitivity reactions (up to 20–30% of patients) [13] or suffer from ‘silent inactivation’ by the neutralizing or opsonizing antibodies [14] , [15] . Modification of ASNase with mPEG in part overcomes these problems [16] , however, a key problem is that antibody responses against mPEG–ASNase continue to occur in ~18% of patients [17] , [18] , [19] . In this study, a molecular sieving pOEGMA coating is optimized for ASNase. In a head-to-head comparison with mPEG–ASNase, pOEGMA–ASNase is ~100-fold less recognized by anti-ASNase antibodies than mPEG–ASNase and 3,000-fold less than the native protein, with a commensurably low loss of activity. In addition, pOEGMA extends the circulation time of ASNase even in mice previously sensitized to ASNase. The semi-permeability characteristics of the coatings are consistent with the phase diagram of protein-bound pOEGMA, which demonstrates that one can design optimal pOEGMA coatings for proteins with little trial-and-error. Polymer architecture, via the comb-shaped nature of pOEGMA, is a potent parameter for optimizing the bioactivity of therapeutic proteins. Molecular sieving pOEGMA–ASNase bio-conjugates ASNase, Fig. 1a , is a tetrameric protein that possesses four identical catalytic sites that transform L -asparagine (Asn) into L -aspartic acid (Asp). As seen in Fig. 1 , the solvent-exposed amino groups (lysine and N -termini in red) are uniformly distributed on the surface of the protein and were converted into initiators for atom transfer radical polymerization. Three ASNase macro-initiators bearing on average x =24, 32 and 36 initiators per protein tetramer were obtained. The degree of modification was assessed by matrix-assisted laser desorption/ionization–time of flight mass spectrometry, which showed symmetric distributions near ~35 kDa (ASNase disassembles into its monomeric form in this experiment; Fig. 1b ). The centre of these distributions was taken as the average degree of modification and correlated well with the feed ratios of reactants ( Supplementary Fig. 1 ). Assuming ASNase to be a sphere with a 3.4-nm radius [20] , these values of x were targeted based on the expectation that a polymer density of at least one pOEGMA chain per ~4 nm 2 of protein surface is required to observe the sieving effect [12] . The polymerization of an OEGMA monomer with eight to ten oxyethylene units was initiated from these sites. Growing polymers directly from proteins is a powerful approach for generating complex bio-conjugates [21] , [22] , [23] , [24] , [25] and offers the advantage of producing a series of comparable bio-conjugates differing uniquely in the length of the polymer backbone ( n ). The length of the polymer backbone was varied by allowing the polymerizations to proceed for different times between 30 min and 4 h. The 19 unique bio-conjugates obtained showed monomodal size-exclusion chromatograms ( Fig. 1c ). 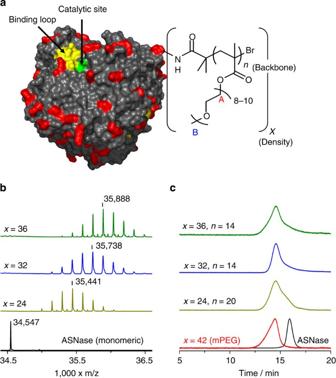Figure 1: Preparation of well-defined pOEGMA–ASNase conjugates. (a) Tetrameric ASNase possesses 92 amino groups (lysine residues and N-termini in red) that are evenly distributed on the solvent-exposed surface of the protein. Nineteen unique pOEGMA–ASNase conjugates were prepared by activation of a certain number (x) of these amino groups with 2-bromoisobutyryl bromide, followedin situgrowth of different length (n) pOEGMA chains by atom transfer radical polymerization. (b) Analysis of the molecular weight of ASNase macro-initiators by matrix-assisted laser desorption/ionization–time of flight mass spectrometry to determine the average number of initiating groups per protein. (c) Representative size-exclusion chromatograms of pOEGMA–ASNase conjugates, mPEG–ASNase and native ASNase. All conjugates tested displayed monomodal molecular-weight distributions. The molecular weight characteristics of the pOEGMA chains were determined by three complementary methods and can be found in Supplementary Table 1 . One ASNase conjugate bearing ca 42 chains of mPEG (5 kDa), determined by 1 H NMR spectroscopy ( Supplementary Fig. 2 ), was produced for comparison. This grafting ratio is in the range expected of commercially available mPEG–ASNase conjugates (Sigma-Aldrich). Figure 1: Preparation of well-defined pOEGMA–ASNase conjugates. ( a ) Tetrameric ASNase possesses 92 amino groups (lysine residues and N-termini in red) that are evenly distributed on the solvent-exposed surface of the protein. Nineteen unique pOEGMA–ASNase conjugates were prepared by activation of a certain number ( x ) of these amino groups with 2-bromoisobutyryl bromide, followed in situ growth of different length ( n ) pOEGMA chains by atom transfer radical polymerization. ( b ) Analysis of the molecular weight of ASNase macro-initiators by matrix-assisted laser desorption/ionization–time of flight mass spectrometry to determine the average number of initiating groups per protein. ( c ) Representative size-exclusion chromatograms of pOEGMA–ASNase conjugates, mPEG–ASNase and native ASNase. All conjugates tested displayed monomodal molecular-weight distributions. Full size image To characterize the molecular sieving characteristics of the conjugates, the conformation of pOEGMA was analysed by 1 H NMR spectroscopy ( Fig. 2a,b ) and correlated to the catalytic activity of the conjugates (aspartyl transferase assay; Fig. 2c ) and their anti-ASNase-binding affinity (sandwich ELISA; Fig. 2d ). As a comb-shaped polymer, pOEGMA can adopt either an ellipsoidal or a cylindrical shape as a function of increasing backbone length n (ref. 26 ). These two states result from the backbone being either in an collapsed or in an extended conformation, a parameter that can be probed by 1 H NMR spectroscopy via peaks ‘A’ and ‘B’ ( Figs 1a and 2a ). As ‘A’ is in close proximity to the polymer backbone ( Fig. 1a ), its integrated value, which becomes less than expected in a rigid un-solvated environment, can be used to estimate its mobility. For this, a reference mobile and solvent-exposed group whose integral is expected to be least affected by de-solvation of the main-chain, such as ‘B’, is required ( Fig. 2a ). Indeed, Roth et al. have shown that ‘B’ retained >92% of its integrated value during pOEGMA’s soluble-to-insoluble transition in alcohol, whereas peak ‘A’ was strongly affected [27] . Herein, peak ‘B’ remained sharp over a wide range of n (12–48; Supplementary Fig. 3 ). 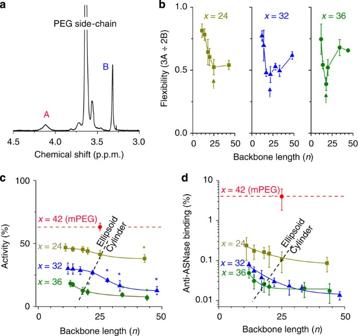Figure 2: Molecular sieving characteristics of pOEGMA–ASNase conjugates. (a) Representative1H NMR spectrum of a pOEGMA–ASNase conjugate with peaks corresponding to ‘A’ and ‘B’ fromFig. 1aidentified. (b) Analysis of the flexibilityFof the pOEGMA backbone permits the identification of the transition between ellipsoidal to cylindrical at the local minimum of the curve (arrow). (c,d) Enzymatic activity and anti-ASNase-binding affinity of ASNase–polymer conjugates, both relative to native ASNase, plotted as a function of polymer backbone lengthn. Inc, star symbols indicate that the measured activity is statistically different from the value at lowestn(ANOVA, TukeyP=0.05;Supplementary Table 2). The sigmoidal curve fit (c) and single exponential decay (d) used to fit the data are to guide the eye. mPEG–ASNase is shown as a line and a symbol in the centre of the graph for ease of comparison. Mean±s.d. (n=3). Figure 2b plots the dimensionless flexibility factor F , calculated from A and B ( F =3A÷2B), which varies between 1 when the backbone is fully solvated and flexible to 0 when it is un-solvated and rigid. The abrupt decrease of F followed by an increase as a function of n is characteristic of protein-bound pOEGMA undergoing an ellipsoid-to-cylinder transition. The increase at high n is observed because F reflects the average flexibility of the entire polymer chain, which increases as it extends away from the protein. The transition, identified by arrows in Fig. 2b , is then projected as a dashed line in Fig. 2c,d , which plot catalytic activity and anti-ASNase-binding affinity, respectively, as a function of x and n . Optimal molecular sieving characteristics were previously observed at n just below the transition between these two conformations [12] . Compared with the first values measured at low n , no statistically significant difference in the catalytic activity of the bio-conjugates was observed in the ellipsoidal regime. A decrease was then observed beyond the transition ( Fig. 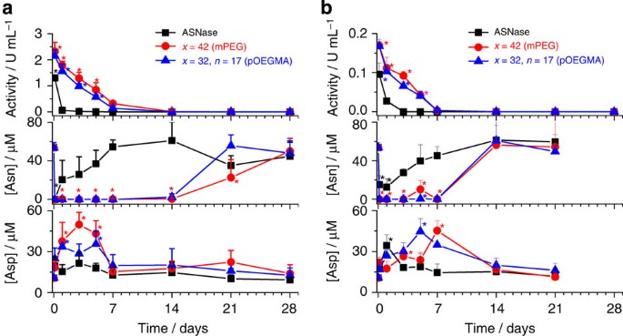Figure 3: Pharmacokinetics of ASNase and ASNase bio-conjugates. (a) 800 IU kg−1or (b) 80 IU kg−1of ASNase, mPEG–ASNase or pOEGMA–ASNase were administered and the catalytic activity,L-asparagine (Asn) concentration andL-aspartic acid (Asp) concentration monitored in blood samples taken at different intervals. The ASNase bio-conjugates showed similar profiles demonstrating that pOEGMA can convey long circulation to proteins, despite being in a compact conformation. Mean+s.d.,n=3. Stars denote statistically significant differences with respect to the natural ASNase activity of blood or to the initial concentration of Asn or Asp (Tukey,P≪0.05). When data points are superimposed, only a single star is shown for clarity. 2c ; full analysis of variance (ANOVA) table in Supplementary Table 2 ; fitted parameters in Supplementary Table 3 ). Shielding of epitopes, assayed via the ability of anti-ASNase antibodies to bind the conjugates, followed a single exponential decay with n ( Fig. 2d ; fitted parameters in Supplementary Fig. 4 ). Increasing the complexity of the fit to a double exponential did not improve the quality of the fit. The rate of decay was more pronounced at higher x , although no obvious manifestation of the change of conformation of pOEGMA was evident in these curves. In comparison to native ASNase, mPEG–ASNase was 1.5 times less catalytically active and 25-fold less recognized by anti-ASNase antibodies. A pOEGMA–ASNase conjugate with optimal semi-permeability characteristics ( x =32, n =17) was only three times less active than the native protein, but was 3,000-fold less recognized by anti-ASNase. Thus, in relation to the small decrease of activity observed between the mPEG and pOEGMA bio-conjugates, the gain in epitope shielding in vitro , and potential for lower immunogenicity in vivo ( vide infra ), is enormous. This pOEGMA–ASNase conjugate ( x =32, n =17) was selected for in vivo analysis because it offered the best compromise between loss of catalytic activity and efficient epitope shielding ( Fig. 2c,d ). Figure 2: Molecular sieving characteristics of pOEGMA–ASNase conjugates. ( a ) Representative 1 H NMR spectrum of a pOEGMA–ASNase conjugate with peaks corresponding to ‘A’ and ‘B’ from Fig. 1a identified. ( b ) Analysis of the flexibility F of the pOEGMA backbone permits the identification of the transition between ellipsoidal to cylindrical at the local minimum of the curve (arrow). ( c , d ) Enzymatic activity and anti-ASNase-binding affinity of ASNase–polymer conjugates, both relative to native ASNase, plotted as a function of polymer backbone length n . In c , star symbols indicate that the measured activity is statistically different from the value at lowest n (ANOVA, Tukey P =0.05; Supplementary Table 2 ). The sigmoidal curve fit ( c ) and single exponential decay ( d ) used to fit the data are to guide the eye. mPEG–ASNase is shown as a line and a symbol in the centre of the graph for ease of comparison. Mean±s.d. ( n =3). Full size image Circulation time and bioactivity of ASNase in vivo Having demonstrated that grafting of pOEGMA did not eliminate catalytic activity, pharmacokinetic experiments were performed. Here 800 IU kg −1 of ASNase, mPEG–ASNase or pOEGMA–ASNase ( x =32, n =17) were administered in saline by intra-peritoneal injection to groups of three BALB/c mice. Blood was withdrawn at regular intervals from the tail vein for analysis of residual ASNase catalytic activity and for analysis of the concentration of Asn and Asp. Native ASNase was rapidly cleared from the body, as evidenced by the complete loss of activity within 1–2 days ( Fig. 3a ). Both mPEG–ASNase and pOEGMA–ASNase displayed sustained activity and depletion of blood Asn below the limit of detection (250 nM) for ca 14 days. At day 21, mPEG–ASNase was the only sample not to have reached its initial Asn concentration. The longer circulation time of mPEG–ASNase is consistent with its slightly larger hydrodynamic diameter (30±5 and 25±5 nm for mPEG–ASNase and pOEGMA–ASNase, respectively) measured by dynamic light scattering. Thus, despite the expected compact conformation of the pOEGMA backbone in its ellipsoidal state, the hydrodynamic volume of the conjugate is sufficient for extended circulation. A transient increase of blood Asp was observed, consistent with the observations of others [28] , indicating that depletion of Asn is occurring according to the expected catalytic mechanism. The observed difference between blood activity and Asn concentration could reflect distribution of the conjugate outside the blood compartment. A lower dose group, receiving 80 IU kg −1 , was also investigated and yielded comparable conclusions ( Fig. 3b ). Figure 3: Pharmacokinetics of ASNase and ASNase bio-conjugates. ( a ) 800 IU kg −1 or ( b ) 80 IU kg −1 of ASNase, mPEG–ASNase or pOEGMA–ASNase were administered and the catalytic activity, L -asparagine (Asn) concentration and L -aspartic acid (Asp) concentration monitored in blood samples taken at different intervals. The ASNase bio-conjugates showed similar profiles demonstrating that pOEGMA can convey long circulation to proteins, despite being in a compact conformation. Mean+s.d., n =3. Stars denote statistically significant differences with respect to the natural ASNase activity of blood or to the initial concentration of Asn or Asp (Tukey, P ≪ 0.05). When data points are superimposed, only a single star is shown for clarity. Full size image Epitope shielding in vivo To assess the efficiency with which the polymers shielded epitopes on ASNase, BALB/c mice were immunized with either ASNase or ASNase bio-conjugates using aluminum hydroxide as adjuvant. Groups of five mice received 20 μg (protein content) of native ASNase, mPEG–ASNase or pOEGMA–ASNase (same conjugates as above) by subcutaneous injections. Analytes were administered on an equal weight (protein) basis to more easily compare their relative ability to generate immune responses. Different results might be expected if the analytes were administered on an equal activity basis, as a lower amount of more active analytes would be administered. For instance, as mPEG–ASNase is twice as active as the selected pOEGMA–ASNase, half as much of it would have been administered. It should also be noted that sensitization was promoted by an adjuvant to test immunogenicity in an accelerated way and that a much lower immune response is to be expected in its absence. Four injections were done with 2-week intervals. Blood was withdrawn on days 28, 42 and 71, and IgG titres towards either ASNase or the bio-conjugate itself were measured. In comparison to the native protein, immunization with mPEG–ASNase and pOEGMA–ASNase conjugates stimulated significantly lower anti-ASNase IgG ( Fig. 4a,b ; orange bars). The results also revealed that immunization with pOEGMA stimulated ~20-fold lower anti-ASNase IgG titres than immunization with mPEG–ASNase, and ~1,000-fold lower than with the native protein. To compare the relative levels of antibodies raised against the conjugates themselves, ELISA plates were coated with mPEG–ASNase or pOEGMA–ASNase ( Fig. 4a,b ; blue bars). The amounts of absorbed native ASNase and ASNase conjugates were verified in order to guarantee that the same amount of protein content was coated into each well, which permits comparisons to be made. On day 28, that is, 2 weeks after the second immunization, low titres of anti-mPEG–ASNase-specific IgG were determined, whereas no pOEGMA–ASNase-specific IgG was detected ( Fig. 4a ). On day 71, 1 month after four immunizations, low conjugate-specific IgG titres were detected for both formulations, but the titre was approximately 20 times lower in serum from mice immunized with pOEGMA–ASNase. Similar results were observed in serum taken on day 42 ( Supplementary Fig. 5 ). These results demonstrate the effectiveness of the comb-shaped polymer in shielding epitopes of ASNase in the adaptive environment of the body. This result is also interesting in light of reports that antibodies can be raised against the polymer component (for example, mPEG) of bio-conjugates and mPEG–ASNase itself [29] , [30] . For robustness, the sensitization experiment was repeated by administrating a higher dose of analyte (200 μg protein per injection) into ASNase-naïve mice according to the same schedule as above. The tenfold increase in ASNase dose resulted in a general three- fourfold increase of IgG titres in all samples analysed, but again with pOEGMA–ASNase producing much lower titres than mPEG–ASNase and native ASNase ( Supplementary Fig. 6 ). 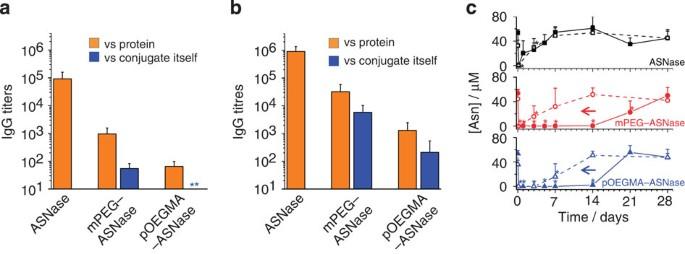Figure 4: Development of new antibodiesin vivo. BALB/c mice were sensitized with either native ASNase, mPEG–ASNase (x=42) or pOEGMA–ASNase (x=32,n=17). (a,b) IgG titres at days 28 and 71. Double stars indicates that signal in undiluted serum was undetectable. (c) Comparison of pharmacokinetic profiles of unsensitized (filled symbols, fromFig. 3a) and sensitized mice administered ASNase and ASNase bio-conjugates on day 72. Mean+s.d. (n=5). Single star denotes statistically significant differences with respect to the natural concentration of Asn (ANOVA, Tukey,P≪0.05). When data points are superimposed, only a single star is shown for clarity. Horizontal arrow indicates shift of the curve because of sensitization. Figure 4: Development of new antibodies in vivo . BALB/c mice were sensitized with either native ASNase, mPEG–ASNase ( x =42) or pOEGMA–ASNase (x=32, n =17). ( a , b ) IgG titres at days 28 and 71. Double stars indicates that signal in undiluted serum was undetectable. ( c ) Comparison of pharmacokinetic profiles of unsensitized (filled symbols, from Fig. 3a ) and sensitized mice administered ASNase and ASNase bio-conjugates on day 72. Mean+s.d. ( n =5). Single star denotes statistically significant differences with respect to the natural concentration of Asn (ANOVA, Tukey, P ≪ 0.05). When data points are superimposed, only a single star is shown for clarity. Horizontal arrow indicates shift of the curve because of sensitization. Full size image Bioactivity of ASNase in ASNase-sensitized mice Long-term treatment with ASNase can produce unwanted antibody responses against the enzyme. This may compromise the biological activity of the therapeutic enzyme. To assess the biological activity of ASNase in such a sensitization model, mice having received the multiple doses of ASNase, mPEG–ASNase or pOEGMA–ASNase according to the schedule above, then received an intra-peritoneal injection of 800 IU kg −1 of the corresponding ASNase formulation 4 weeks after the last of four immunizations. Before injection, Asn concentrations in blood were normal and the sensitizing ASNase preparations had no residual enzymatic activity. As seen in Fig. 4c , neither native ASNase nor mPEG–ASNase were able to maintain full depletion of blood Asn beyond the first 3 h after injection, whereas full depletion was still observed for pOEGMA–ASNase at day 3. Normal Asn levels were observed by day 7 for both native ASNase and mPEG–ASNase and by day 14 for pOEGMA–ASNase. Although the half-lives of both polymer–ASNase conjugates were significantly shorter than those observed in the non-sensitized animals, the longer circulation time of pOEGMA–ASNase vs mPEG–ASNase appears to reflect the lower immune response raised for this conjugate during sensitization and suggests that pOEGMA conveys better stealth-like characteristics to ASNase than does mPEG, even after repeated dosing. The desire to effectively shield enzymes with polymers, without compromising activity, has driven multiple systematic studies in which the influence of grafting density, polymer molecular weight, polymer type (that is, synthetic, natural), coupling chemistry and so on, have been examined [31] , [32] . However, studies that directly compare linear polymers to (related) branched ones are rare. In two important studies, Veronese and co-workers compared the activity, pH and temperature stability, and proteolytic digestion of ASNase (from Erwinia Carotivora ) and three other enzymes modified with either linear mPEG or double-branched mPEG (mPEG 2 ) [33] , [34] . Although, for the most part, catalytic activity was similar for the mPEG and mPEG 2 bio-conjugates, all of the enzymes modified with mPEG 2 were more resistant to proteolysis. This is consistent with the more facile diffusion of small vs large molecules through the polymer coating, as observed herein. Furthermore, the antigenicity of the mPEG 2 –ASNase conjugate was lower than for the mPEG analogue, although the difference was smaller than that observed herein. The present study expands upon these observations and emphasizes how controlling the molecular dimensions of the architecturally complex polymer pOEGMA beneficially reduces the immunogenicity of a subclass of biomolecules with diffusible small molecules as their substrates. Dense pOEGMA coatings are well-known to efficiently repel the adsorption of proteins to solid surfaces, such as gold [35] , [36] . However, the application of this strategy to protect proteins themselves has met little attention. The dissuading dogma is the expected strong negative effect multiple polymer conjugation will have on the protein’s bioactivity because of obstructed interaction with its binding partners, substrates and so on [31] . To our knowledge, Magnusson et al. [37] have presented the only in vivo study of the shielding efficacy of multiple pOEGMA chains on a protein, recombinant human growth hormone. The beneficial properties observed, however, were attributed to enhanced stability and prolonged pharmacokinetic profile, which counterbalanced the expected loss of activity, rather than to an intrinsic characteristic of nonlinear polymers or pOEGMA itself. Of course, the mechanism of action of recombinant human growth hormone involves receptor binding rather than enzymatic activity, which is probably why the relevance of the architecture of pOEGMA was not discussed. Other in vivo studies have focused on extending the circulation half-life of proteins with single pOEGMA chains [38] , [39] , [40] . Thus, the most significant contribution herein is the demonstration of the particularity of pOEGMA, which can be conveniently and rationally manipulated to address the dogma of loss of activity, even in the complex environment in vivo . This is an important finding because many non-human-derived proteins, including ASNase, possess numerous epitopes or enzyme-sensitive segments that can be responsible for treatment failure if they are not adequately shielded [41] , [42] . In fact, as ASNase is a homo-tetrameric protein, all epitopes are present in four identical copies. Thus, this type of protein absolutely requires multiple polymer conjugation because of the inability of a single (or a few) polymer chains to adequately shield these problematic parts of the protein [43] , [44] . Finally, it is worth considering that pOEGMA is attached to the protein via an amide bond and is unlikely to be released from the conjugates within the timeframe of the experiments performed. Ultimately, however, one would expect degradation of ASNase, which would release single pOEGMA chains connected to short peptide segments. Considering the molecular weight of the pOEGMA used (that is, n =17 is ~8 kDa), it should ultimately be eliminated by, for example, renal filtration. In summary, this study is the first in vivo demonstration of how polymer architecture, via the comb-shaped nature of pOEGMA, provides a unique design parameter for optimizing therapeutic proteins. The combined properties of effective epitope shielding with proportionately low loss of activity are inaccessible by conventional ‘PEGylation’ using linear polymers. Using ASNase as a model therapeutic protein, the designed pOEGMA bio-conjugate outperformed the mPEG–ASNase control (of similar catalytic activity) by being less immunogenic and providing a more sustained activity in sensitized animals. This shows promise for long-term therapies involving pOEGMA-modified proteins. Importantly, observations were consistent with predictions made from the phase diagram of protein-bound pOEGMA [12] . This guided the design of optimal semi-permeable coatings alongside convenient spectroscopic analysis of polymer conformation. This implies that one can easily design optimal pOEGMA coatings for proteins with little trial-and-error. One caveat is the limitation to therapeutic proteins that target soluble substrates small enough to penetrate through the pOEGMA coating. This makes the findings above most applicable to enzymes such as asparaginase, methioninase, arginine deiminase, arginase, uricase and so on [32] . Nevertheless, the presented strategy could also be used to protect and alter the circulation lifetime of emerging classes of therapeutics, such as small-molecule-binding proteins that could be used as drug scavengers [45] , and create non-fouling coatings for biosensors that are specific towards small analytes. ASNase pOEGMA–ASNase and mPEG–ASNase E. coli ASNase was purchased from Afine Chemicals Ltd and de-salted before use. The synthesis, purification and characterization of ASNase bio-conjugates follow a robust procedure adapted from the original work of Lele et al. [22] and is described in detail in the Supplementary Methods . In vitro catalytic activity ASNase and ASNase bio-conjugate catalytic activities were assayed by the formation of aspartate hydroxamate from Asn and hydroxylamine (aspartyl transferase activity). 20 μl of a 50 μg ml −1 (protein) aqueous enzyme solution were added to 1 ml Tris-HCl buffer (100 mM, pH 7.4) containing 20 μM Asn and 400 μM hydroxylamine. The mixture was incubated at 37 °C for 30 min, after which 700 μl of ferric chloride agent (5% ferric chloride, 1 M HCl, 4% trichloroacetic acid) were added. Aspartate hydroxamate forms a coloured complex with ferric chloride that can be quantified at 500 nm (ref. 46 ). In vitro recognition by anti-ASNase antibodies Streptavidin-coated 96-well microplates (Pierce) were rinsed with 3 × 200 μl wash buffer (25 mM Tris, 150 mM NaCl, 0.25% bovine serum albumin, 0.05% Tween-20, pH 7.2) after which 100 μl of biotinylated anti-asparaginase antibody (10 μg ml −1 ) wash buffer was added and incubated for 2 h room temperature. The wells were rinsed with 3 × 200 μl wash buffer after which 100 μl of serial dilutions of native ASNase (1 μg ml −1 to 1 pg ml −1 ) were incubated for 30 min at room temperature to obtain a response curve. Thereafter, 100 μl of either mPEG–ASNase or pOEGMA–ASNase (1 μg ml −1 ) were analysed in the same manner and the value compared with this response curve. The wells were rinsed with 3 × 200 μl wash buffer, and 100 μl horseradish peroxidase-labelled anti-asparaginase antibody (4 μg ml −1 in wash buffer) was added and incubated for 30 min. After a final rinse with 6 × 200 μl wash buffer, 100 μl 1-Step Slow TMB-ELISA Substrate Solution was added. After exactly 10 min, 50 μl 2 N HCl was added and absorbance of each well was measured at 450 nm. Pharmacokinetics in naïve mice All animal protocols were approved and conducted according to the guidelines of the Cantonal Veterinary Office Zurich. Groups of three female BALB/c mice (25 g) were administered either 80 or 800 IU kg −1 of ASNase, pOEGMA–ASNase ( x =32, n =17) or mPEG–ASNase ( x =42) in 100 μl sterile saline by intra-peritoneal injection. One international unit (IU) of activity is defined herein as the amount of enzyme that catalyses the formation of 1.0 mmol of Asp per min at 25 °C. Approximately 50 μl blood was sampled from the tail vein repeatedly over 28 days, and was immediately centrifuged for collection of serum that was stored frozen (−80 °C) until analysed. Sensitization and enzymatic activity in sensitized mice Groups of five female BALB/c mice were immunized on days 0, 15, 29 and 43 by subcutaneous injections of 100 μl of a sterile saline solution containing either 20 or 200 μg protein content in ASNase, pOEGMA–ASNase ( x =32, n =17) or mPEG–ASNase ( x =42). All vaccine preparations also contained 0.6 wt% Alhydrogel (Brenntag Biosector). Blood was collected on days 28, 42 and 71 as described above. On day 72, all mice from the low-dose groups were administered 800 IU kg −1 of the corresponding ASNase or ASNase bio-conjugate in 100 μl sterile saline by intra-peritoneal injection, and blood was sampled for measurement of Asn metabolism as described above. Blood analysis Bioactivity of native ASNase and polymer-modified ASNase was measured with an Asparaginase Activity Assay Kit (MAK007, Sigma-Aldrich) according to the manufacturer’s recommended protocol. The concentrations of Asn and Asp in mice serum were analysed using pre-column derivatization high-performance liquid chromatography ( Supplementary Figs 7 and 8 ) according to a method modified from Bidlingmeyer and described in the Supplementary Methods [47] . Blood antibody titres were measured by sandwich ELISA as described in the Supplementary Methods . Statistics Means from activity tests were compared by one-way ANOVA followed by a Tukey post-hoc test. Means from pharmacokinetics data were compared by one-way repeated-measures ANOVA followed by a Tukey post-hoc test. Differences were considered significant at P ≪ 0.05. How to cite this article: Liu, M. et al. Semi-permeable coatings fabricated from comb-polymers efficiently protect proteins in vivo . Nat. Commun. 5:5526 doi: 10.1038/ncomms6526 (2014).